Wave–matter interactions in epsilon-and-mu-near-zero structures In recent years, the concept of metamaterials has offered platforms for unconventional tailoring and manipulation of the light–matter interaction. Here we explore the notion of ‘static optics’, in which the electricity and magnetism are decoupled, while the fields are temporally dynamic. This occurs when both the relative effective permittivity and permeability attain near-zero values at a given operating frequency. We theoretically investigate some of the resulting wave features in bounded scenarios, such as unusual radiation characteristics of an emitter embedded in such epsilon-and-mu-near-zero media in bounded environments. Using such media, one might in principle ‘open up’ and ‘stretch’ the space, and have regions behaving electromagnetically as ‘single points’ despite being electrically large. We suggest a possible design for implementation of such structures using a single dielectric rod inserted in a waveguide operating near its cutoff frequency, providing the possibility of having electrically large ‘empty’ volumes to behave as epsilon-and-mu-near-zero media. Throughout the last decade, there have been extensive research efforts in the field of metamaterials [1] , [2] , [3] , [4] , [5] —artificial structures that exhibit unusual properties that do not readily exist in nature. Recently, there has been great interest in the near-zero-parameter materials. This is the category of metamaterials whose relative permittivity is near zero (that is, epsilon-near-zero (ENZ)), or relative permeability is near zero (that is, mu-near-zero (MNZ)), or both relative permittivity and permeability are near zero (that is, epsilon-and-mu-near-zero (EMNZ)). The special feature of such media basically lies in having a low wave number (that is, stretched wavelength) as a consequence of the near-zero refractive index that leads to a relatively small phase variation over physically large region of such media. This has opened the door to various interesting wave phenomena and applications. One track in which this category of metamaterials was utilized efficiently is the field of antenna design, where ENZ or EMNZ materials were considered for tailoring the radiation patterns, that is, to attain highly directive radiation patterns [6] , [7] , [8] , [9] , [10] , [11] , [12] , or for significantly enhancing the radiation efficiency [13] , [14] , [15] . On the other hand, near-zero-parameter materials have also been extensively studied and used as means to realize unconventional tunnelling of electromagnetic energy within ultrathin subwavelength ENZ channels or bends (a phenomenon coined as supercoupling) [16] , [17] , [18] , [19] , tunnelling through large volumes using MNZ structures (Marcos, J. S, Silveirinha, M. & Engheta, N., manuscript in preparation), and to overcome the problem of weak coupling between different electromagnetic components that are conventionally not well matched, for example, in a coaxial to waveguide transition [20] . Another interesting field of research has been about manipulating the transmission characteristics using near-zero media [21] , [22] , [23] , [24] where such media have been loaded by certain properly designed inclusions that allow shaping of the system’s transmission profile. Recently, the field of anisotropic near-zero-parameter media has also been explored, adding extra degrees of freedom and thus achieving some interesting phenomena [25] , [26] , [27] , [28] . Moreover, zero parameter materials have been integrated with nonlinear elements to achieve controllable transmission [29] or to enhance the nonlinear response of Kerr-based structures in the optical regime [30] , [31] . Owing to the numerous potential applications and novel physical phenomena that can result from such media, great efforts have been put into the actual realization of those media, from naturally available materials [32] , [33] , [34] to using photonic crystals that exhibit dirac cone dispersion [35] , [36] and structures in the microwave regime [37] , [38] , and suggestions for the more challenging optical regime [39] , [40] , [41] where gain media has usually been exploited to overcome the problem of high losses [41] . It is also worth mentioning here the research efforts related to the so-called DB boundary conditions, namely the set of boundary conditions that require vanishing normal components of D and B vectors at the interface. Within that context, reflection of arbitrary plane waves was analysed for the planar DB boundary as described in ref. 42 and it was shown that transverse electric (TE) and transverse magnetic (TM) waves are reflected from respective perfect electric conductor and perfect magnetic conductor planes [42] . Moreover, possible realizations of the DB boundary in terms of an interface of uniaxially anisotropic metamaterial half-space with zero axial parameter media or sheets have also been studied by the same authors [42] , [43] , [44] . However, in those lines of work the main emphasis was on plane waves with oblique incidence angles, showing that such interfaces can act as spatial filters reflecting plane waves incident at any angle for both polarizations with the exception of a narrow window around normal incidence. In the present work, we shed light on some of the other exotic phenomena of EMNZ media in bounded scenarios, providing a study regarding two of the main pillars of electromagnetic behaviour within EMNZ-bounded environments, namely its scattering properties and its interaction with emitting dipoles. Moreover, building on the findings in earlier lines of work [17] we propose a design scheme that provides us with both effective permittivity and effective permeability near zero over a relatively large ‘empty’ volume, and discuss the limitations. Opening up the space Since in such an EMNZ medium, both ∇ × E =0 and ∇ × H =0 simultaneously, the electric and magnetic phenomena are decoupled and spatially distributed statically, while still temporally dynamic [10] . This leads to a paradigm in which we may have optical phenomena, while the field distributions are static-like, effectively having a scenario as ‘DC optical circuits’. Having such an EMNZ region, as shown in Fig. 1a , we can break an air-filled parallel-plate waveguide at a point, and effectively ‘open up’ or ‘stretch’ the space between two parts of this waveguide, without affecting external electromagnetic entities and quantities, implying that we can have an electromagnetically large bounded physical volume, that would have otherwise influenced the electromagnetic wave propagation externally, but now owing to the EMNZ effect it behaves as if it is a ‘single point’ electromagnetically as viewed from the external world. The external boundary of the entire two-dimensional (2D) region shown in Fig. 1 (except for the input and output exit ports) is perfectly electric conducting (PEC) wall. As depicted in a 2D simulation shown in Fig. 1b , perfect transmission (with unit magnitude and zero phase difference) from the input to the output port is preserved regardless of the arbitrary shape and size of the EMNZ region. Moreover, in this 2D simulation of the EMNZ region, the magnetic field spatial distribution is uniform, while the electric field is distributed spatially as though a ‘battery’ is connected between the top and the bottom plates of the EMNZ region. 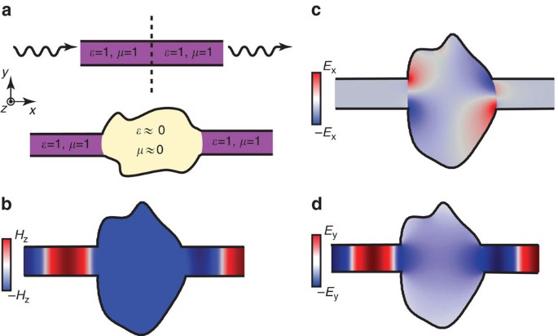Figure 1: EMNZ medium as an ‘electromagnetic point’. (a) Schematic of an EMNZ medium emulating opening up or stretching the space at the dotted line between the two sections of an air-filled parallel-plate waveguide, while keeping the region as a ‘single point’ electromagnetically. (b) Snapshot of thez-component of the magnetic field distribution (shown with colour map) and thex-component (c) andy-component (d) of the electric field distributions over the proposed 2D structure with an arbitrarily shaped cross-section filled with an idealized EMNZ material. The external walls (except at the exits of the two ports) are made of PEC. Figure 1: EMNZ medium as an ‘electromagnetic point’. ( a ) Schematic of an EMNZ medium emulating opening up or stretching the space at the dotted line between the two sections of an air-filled parallel-plate waveguide, while keeping the region as a ‘single point’ electromagnetically. ( b ) Snapshot of the z -component of the magnetic field distribution (shown with colour map) and the x -component ( c ) and y -component ( d ) of the electric field distributions over the proposed 2D structure with an arbitrarily shaped cross-section filled with an idealized EMNZ material. The external walls (except at the exits of the two ports) are made of PEC. Full size image Scattering within EMNZ media An interesting phenomenon that takes place within EMNZ-bounded environments is the unconventional scattering performance of PEC objects embedded in an EMNZ medium. Recently, there has been some lines of work investigating the behaviour of zero-index media when loaded by various structures and the ability of these systems to manipulate the transmission and reflection profile owing to the unique scattering performance within zero-index media [21] , [22] , [23] , [24] . Here using the 2D Mie scattering theory we study the unique scattering performance from 2D PEC objects, embedded in a 2D host EMNZ medium. We begin by analytically solving for the scattered fields from a 2D PEC cylinder of radius a embedded in an unbounded EMNZ medium for both the TM (that is, the incident H vector is parallel with the cylinder axis) and TE (that is, the incident E vector is parallel with the cylinder axis) incident waves normally incident on the cylinder. For a TM wave, the incident and the scattered fields can be written (assuming e − iωt and that the axis of the cylinder is along the z axis) in the time-harmonic case as follows Applying the boundary conditions we find that Similarly, for the TE case, we can find that We investigate the dependence of |C n | on k EMNZ as depicted in Fig. 2a,b . As shown, there exists an interesting difference between the scattering behaviour of the cylinder being illuminated by a TM wave versus a TE wave. For the TM mode as shown in Fig. 2a the dependence of |C n | on k EMNZ is relatively weak around the strict zero condition, meaning that for the case where k EMNZ is small but not strictly zero we can still consider having zero |C n | for all n ’s. Thus, for that mode a conducting cylinder would introduce no scattering and would be totally cloaked. (An intuitive way to appreciate this point is to consider the fact that in the EMNZ medium, D =0, and thus ∇ · D =0. Therefore, no charge can be induced on the surface of this 2D PEC cylinder when illuminated by the TM wave.). On the other hand, Fig. 2b shows that for the TE mode |C 0 | exhibits a relatively stronger dependence on k EMNZ in vicinity of the strict zero condition, suggesting that for the case where k EMNZ is near zero, but not strictly zero, we should expect a strictly non-zero scattering from the cylinder with the scattered fields being azimuthally symmetric, when illuminated by that mode. These findings are verified numerically in the insets of Fig. 2a,b where in (a) we see the scattered fields from a PEC cylinder of radius 5 λ 0 , with λ 0 being the free space wavelength, embedded in an EMNZ-unbounded medium, and illuminated by a TM wave. As expected, the scattered fields because of the 2D PEC cylinder vanish. On the other hand, the inset of Fig. 2b shows the scattered fields from a conducting cylinder of the same radius that is illuminated by a TE wave. It is shown that for that polarization we get a non-zero scattering only for the n =0 component of the scattered field when the relative permittivity and permeability are near zero (but not strictly zero), as expected. Moreover, the interesting property of PEC objects introducing no scattering being illuminated by a TM wave when embedded in an EMNZ medium still holds regardless of how arbitrarily shaped the EMNZ region and the conducting object are, owing to the ability of EMNZ media to open up the space as discussed before. This is depicted clearly in Fig. 2c , where a physically large-cross-section 2D PEC cylinder of an arbitrary shape is embedded into the EMNZ-bounded region with another arbitrary shape connected to two air-filled parallel-plate waveguides, shown in Fig. 1b , providing no scattering at all, with unity transmission and almost no phase progression as the wave traverses the EMNZ region containing this cylinder. (As in Fig. 1 , the external boundary (except for the input and output ports) is made of PEC wall. The two parallel-plate waveguides connected to the 2D EMNZ region are filled with air.). 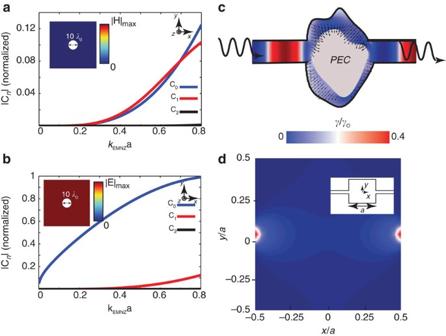Figure 2: Mie scattering coefficients and spontaneous emission rate in EMNZ. Mie scattering coefficients for (a) TM mode and (b) TE mode. 2D scattered magnetic field from a 2D conducting cylinder of radius 5λ0embedded in an ideal EMNZ medium when illuminated by TM mode (inset (a)), and 2D scattered electric field from a conducting cylinder of radius 5λ0embedded in an ideal EMNZ medium when illuminated by TE mode (inset (b)). (c) Snapshot of the 2D electric (shown as arrows) and magnetic (shown as colour map) field distributions in a 2D EMNZ region, loaded with a conducting cylinder, both with arbitrarily shaped cross-sections. External walls (other than the exits of the two ports) are assumed to be PEC walls. (d) Distribution of normalized spontaneous emission rate of a 2D electric dipole inside the 2D EMNZ enclosure with two ports connected to parallel-plate waveguides filled with air versus the dipole position within the structure. The geometry of the EMNZ enclosure and the two air-filled parallel-plate waveguides are shown in the inset. Figure 2: Mie scattering coefficients and spontaneous emission rate in EMNZ. Mie scattering coefficients for ( a ) TM mode and ( b ) TE mode. 2D scattered magnetic field from a 2D conducting cylinder of radius 5 λ 0 embedded in an ideal EMNZ medium when illuminated by TM mode (inset ( a )), and 2D scattered electric field from a conducting cylinder of radius 5 λ 0 embedded in an ideal EMNZ medium when illuminated by TE mode (inset ( b )). ( c ) Snapshot of the 2D electric (shown as arrows) and magnetic (shown as colour map) field distributions in a 2D EMNZ region, loaded with a conducting cylinder, both with arbitrarily shaped cross-sections. External walls (other than the exits of the two ports) are assumed to be PEC walls. ( d ) Distribution of normalized spontaneous emission rate of a 2D electric dipole inside the 2D EMNZ enclosure with two ports connected to parallel-plate waveguides filled with air versus the dipole position within the structure. The geometry of the EMNZ enclosure and the two air-filled parallel-plate waveguides are shown in the inset. Full size image Dipole emission within EMNZ media In this section we investigate the behaviour of emitting dipoles within arbitrarily shaped EMNZ media, and more specifically how the EMNZ environment influences the spontaneous emission rate of emitters leading to some interesting unprecedented behaviour. In ref. 16 the phenomenon of supercoupling that relies on energy squeezing through subwavelength narrow channels has been introduced in ENZ metamaterials. Owing to the substantial electric field enhancement within the narrow ENZ channel, placing an electric-dipole emitter within that ENZ channel leads to significant emission enhancement that can be quantitatively described in terms of the dipole’s spontaneous emission rate γ as compared with its emission rate in free space γ o , that is, γ / γ o (refs 18 , 45 ). However, a unique feature of such structure as compared with any other resonant system coupled to a radiating element or molecule is the nearly uniform phase distribution of that enhanced electric field along the channel, which is in principle independent of the channel length. This leads to the independence of the emission enhancement on the dipole’s location within the channel [18] , [45] . In an EMNZ medium on the other hand, the supercoupling phenomenon is still preserved, however, without the need for ultranarrow subwavelength channels as was the case for ENZ media, which in addition to providing a larger platform to place the dipole within the medium, leads to no mandatory enhancement in the fields within the EMNZ region. This may lead to the novel effect of emission inhibition regardless of the position of the dipole within the EMNZ region. To numerically demonstrate that phenomenon, we investigate the 2D structure shown in the inset of Fig. 2d , where a 2D y -oriented dipole is placed within a 5 λ 0 × 5 λ 0 bounded enclosure filled with an ideal EMNZ material connected to two narrow parallel-plate waveguides filled with air. (The cross-sectional shape of this 2D EMNZ region is chosen arbitrarily. The external boundary, except for the two ports, is made of PEC wall.). As shown in Fig. 2d where a colour map of 2D distribution of γ / γ o versus the dipole location within the EMNZ region is shown, we get significant emission inhibition (that is, γ / γ o less than unity) within the EMNZ region as expected. Owing to the reciprocity, this γ / γ o distribution resembles the distribution of the y- component of the electric field when this structure is fed with the transverse electromagnetic mode incident from one of the air-filled parallel-plate waveguide ports. Now we explore a scenario in which a properly selected single dielectric inclusion within a host medium whose permittivity (or effective permittivity) is near zero (for example, a large waveguide section with the TE 10 mode near its cutoff frequency) [46] may lead to simultaneously have effective permittivity and permeability near zero. We also explore the limits to which such a structure could mimic the interesting characteristics discussed in the previous sections, including the ability to open up the space, the unique scattering performance of electrically large PEC structures embedded in it and nonconventional radiation performance for radiating elements placed within the proposed structure. It was shown in previous work [17] that with an ENZ host medium one can also achieve an effective MNZ by periodically loading this host medium with inclusions of proper dimensions and permittivity. In this section we show that this can be extended into a nonperiodic case with arbitrary shape of the cross-section, and that even within one unit cell, which can be arbitrarily large and not limited to a subwavelength size, we can still have both effective permittivity and permeability near zero. We propose a practical design in which the interesting features of EMNZ can be studied in the microwave regime. At such frequencies, ENZ materials are not readily available in nature; however, it has been shown in ref. 47 that parallel metallic plates can simulate a 2D artificial plasma when the TE 10 mode is considered. The effective permittivity of the such waveguide structures follows a Drude-like model, that is, ε h / ε 0 = ε d −( π / k 0 d ) 2 , where ε d is the relative permittivity of the dielectric between the metallic plates, d is the separation between the metallic plates and k 0 is the wave number in free space. In such an environment, if d is chosen to be λ 0 /2, where λ 0 is the free space wavelength at some chosen operating frequency ω c we need to load this waveguide with a material of permittivity ε i +1, in order to emulate a material with relative permittivity ε i . Thus, as shown in Fig. 3a the input and output channels that are required to emulate an air-filled parallel-plate waveguide with the transverse electromagnetic mode are mimicked using TE 10 mode in rectangular waveguides filled with a dielectric of relative permittivity of 2 (regions 1 and 3). In the proposed EMNZ region (region 2 in the middle) the ENZ host medium is emulated by a waveguide filled with dielectric of relative permittivity of 1. We choose the inclusion to be a circular-cylinder dielectric rod of radius R and permittivity ε i by which, when embedded periodically in an ENZ host, one can achieve an effective permeability shown in ref. 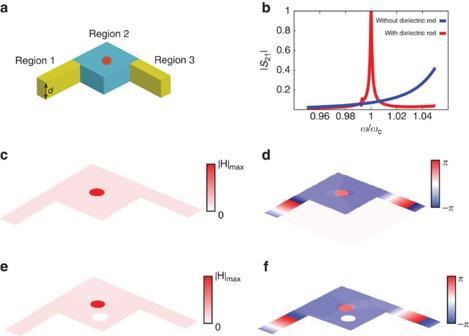Figure 3: Proposed design for a structure imitating effectively an EMNZ medium. (a) Geometry of rectangular air-filled metallic waveguide structure (middle region, blue) with a dielectric rod inclusion (red) emulating the EMNZ behaviour. This middle section is connected to two identical dielectric-filled metallic rectangular waveguides (yellow) as the two ports. (b) Magnitude of the transmission coefficient (S21) of the structure shown inaversus normalized frequency, when fed by one of the waveguide ports. Hereωcis the cutoff radian frequency of the waveguide section. Red and blue curves are for the cases of with and without the dielectric rod, respectively. (c) Amplitude and (d) phase of the magnetic field in the middle plane within the structure, when it is illuminated by a wave coming from one of the ports. (e,f) Amplitude and phase of the magnetic field in the middle plane within the structure when the PEC scattering cylinder is also inserted. 17 to be Figure 3: Proposed design for a structure imitating effectively an EMNZ medium. ( a ) Geometry of rectangular air-filled metallic waveguide structure (middle region, blue) with a dielectric rod inclusion (red) emulating the EMNZ behaviour. This middle section is connected to two identical dielectric-filled metallic rectangular waveguides (yellow) as the two ports. ( b ) Magnitude of the transmission coefficient ( S 21 ) of the structure shown in a versus normalized frequency, when fed by one of the waveguide ports. Here ω c is the cutoff radian frequency of the waveguide section. Red and blue curves are for the cases of with and without the dielectric rod, respectively. ( c ) Amplitude and ( d ) phase of the magnetic field in the middle plane within the structure, when it is illuminated by a wave coming from one of the ports. ( e , f ) Amplitude and phase of the magnetic field in the middle plane within the structure when the PEC scattering cylinder is also inserted. Full size image where A cell is the total area ( a × a ) of the unit cell, A h ,cell = A cell − πR 2 , and . (Note that this rod can be placed almost anywhere in the unit cell. Moreover, although in Fig. 3a the cross-section of the middle section is taken to be rectangular, any arbitrary shape with the required area can be chosen.) As mentioned before, we are interested in a near zero-effective permeability, which for a =1.3 λ 0 with a dielectric rod of radius 0.13 λ 0 requires the rod’s relative permittivity to be 9.82. We show that even using only one unit cell we still get almost perfect transmission at the operating frequency ω c as numerically shown in Fig. 3b as opposed to getting almost no transmission in absence of the dielectric rod. Figure 3c shows a cross-section of the distribution of the magnitude of the magnetic field within the structure, and the almost perfect transmission between the two ports is evident here, with almost uniform phase within the proposed EMNZ region as shown in Fig. 3d . Thus, it is numerically verified that our proposed structure acquires the desired EMNZ behaviour of opening up the space with near unity magnitude and zero phase transmission between the two ports. Intuitively, the presence of the dielectric rod, when designed properly, generates enough magnetic field inside the rod mostly in the opposite direction to the magnetic field in the ENZ region (that is, outside the rod) in order to make the total flux of μ 0 H to reach zero, achieving an effective near-zero permeability. The above design with the PEC walls is suitable for the microwave frequencies, in which highly conductive materials are readily available. However, in the optical regime, the metallic walls are lossy. The effect of this loss and an alternative design using the photonic bandgap dielectric structures as the walls suitable for the optical frequencies are discussed in Supplementary Note 1 and 2 . It is worth mentioning that a small amount of mode coupling from the original TE 10 mode to the TM 10 mode may occur due to the curved boundary of the rod’s cross-section in the middle structure, since these two modes have the same cutoff frequencies in the parallel-plate waveguides. However, such small mode coupling may be reduced by adding few tiny conducting wires around the dielectric rod. This is the subject of our ongoing study and will be reported in a future publication. Next, we proceed to investigate whether having a PEC cylinder embedded in our proposed effectively EMNZ structure would introduce no scattering for the incident mode with the magnetic field vector parallel with the axis of the cylinder as discussed previously. This is depicted clearly in Fig. 3e,f where a PEC cylinder of radius 0.13 λ 0 is embedded into the proposed structure. It is worth mentioning here that now loading the EMNZ unit cell with a conducting cylinder, the effective area of the unit cell is reduced, and that consequently for the same radius of a dielectric rod, the rod’s permittivity has to be adjusted to take that into account. As depicted clearly in Fig. 3e,f , the conducting rod does not introduce any scattering as expected. Finally, we investigate an electric-dipole emission performance within our proposed structure. The phenomena of opening up the space and the unique scattering performance within an EMNZ medium are effectively ‘global’ phenomena, that is, they can be described using effective media approaches. On the contrary, the dipole spontaneous emission rate is a phenomenon that is highly dependent on its surrounding environment. Thus, one might expect the spontaneous emission inhibition phenomenon that was shown previously within an idealized EMNZ medium would not necessarily take place within our proposed structure, whose ‘effective’ permittivity and permeability exhibit near-zero values (while the local material parameters may differ from zero), but the radiation from the ports may be influenced by such effective EMNZ characteristics. We numerically examine the radiation of a given x -oriented short electric dipole placed in various locations inside our proposed design for the effectively EMNZ-bounded structure with two ports to the outside region. As shown in Fig. 4a , where γ / γ o distribution as a function of the dipole’s location within the proposed structure is given, there exists a significant enhancement in the spontaneous emission rate of such a dipole when it is located in proper locations within the structure. This enhancement is more pronounced towards the centre of the structure, completely consistent with reciprocal scenario when one would get high values of electric field near the dielectric rod, if the incident energy was fed as a TE 10 mode through one of the waveguide ports. This can also be explained by noting that as the dipole gets closer to the centre, the fundamental mode of the dielectric rod (that is, the mode for which effective zero permeability is achieved) is better coupled to the dipole emission. One of the highlights of the dipole emission in such an effectively EMNZ structure is the intriguing phenomenon of the equal distribution of the radiated power between the two output ports (due to the uniformity of the phase within the structure), regardless of the relative location of the dipole to either of the ports and regardless of the location of the ports connected to the structures. This is shown in Fig. 4b–d where moving the dipole from the centre to the corner or towards the left port does not introduce any change on the ratio between the powers exiting the two ports. Specifically, while the total radiated power from the dipole may depend on its location inside this structure (for example, this total power is weaker in Fig. 4c,d than in Fig. 4b ), this power is divided equally as it exits from the two ports when the two ports’ cross-sections are the same. This intriguing power division is independent of how close the dipole may be located near one of the ports and is also independent of where the two ports are connected to the structure. As can be seen in Fig. 4d , the waves exiting from the two ports are the same (with the same amplitude and phase), even though the dipole is very close to the left port and far from the right port. This implies that the radiation from the dipole couples to the two ports the same way, despite unequal distance of the dipole from the two ports. This phenomenon may have important implications in quantum optics and the photon entanglement in such platforms. We will report on this issue in a future publication. 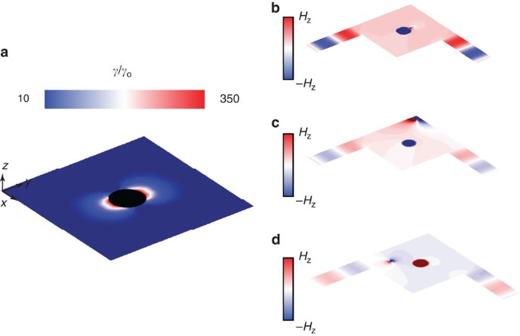Figure 4: Emission of a dipole located inside the proposed structure. (a) Distribution of the normalized spontaneous emission rate of thex-oriented short electric dipole versus the dipole position within the designed enclosure imitating EMNZ medium. (b) A snapshot of the magnetic field of the dipole radiation within the structure with the short electric dipole placed close to the centre. Panelcas inb, but the dipole is brought to the corner of the structure. Paneldas inb, but the dipole is brought close to the left port. While the total radiated power is different inb–d, the power exited from the two ports is divided equally in each case, regardless of the location of the dipole within the structure and the relative location of the dipole to the ports. Figure 4: Emission of a dipole located inside the proposed structure. ( a ) Distribution of the normalized spontaneous emission rate of the x -oriented short electric dipole versus the dipole position within the designed enclosure imitating EMNZ medium. ( b ) A snapshot of the magnetic field of the dipole radiation within the structure with the short electric dipole placed close to the centre. Panel c as in b , but the dipole is brought to the corner of the structure. Panel d as in b , but the dipole is brought close to the left port. While the total radiated power is different in b – d , the power exited from the two ports is divided equally in each case, regardless of the location of the dipole within the structure and the relative location of the dipole to the ports. Full size image In conclusion, we have explored some of the intriguing phenomena of dipole emission and wave scattering in EMNZ-bounded structures, and have proposed a design using a single dielectric rod embedded in a metallic waveguide near its TE 10 cutoff frequency, imitating the medium with both effective relative permittivity and permeability near zero. We have numerically shown that this design exhibits the relevant features of the EMNZ structures. The numerical results shown in Figs 1 , 2c,d and 4 were achieved using the RF module of the finite-element-method commercial software COMSOL Multiphysics, using triangular meshing of maximum element size λ 0 /30, where λ 0 is the operating wavelength in free space. The numerical results shown in Fig. 3 were performed using the time domain solver of the commercial software CST Microwave Studio, using automatic meshing. For the normalized spontaneous emission rate calculations shown in Figs 2d and 4a , a point dipole emitter has been used whose dipole moment has been fixed and for each location the total radiated power was calculated numerically from which the corresponding spontaneous emission rate can be found analytically and normalized to the spontaneous emission rate of the same dipole moment at the same frequency in free space. How to cite this article : Mahmoud, A. M. and Engheta, N. Wave–matter interactions in epsilon-and-mu-near-zero structures. Nat. Commun. 5:5638 doi: 10.1038/ncomms6638 (2014).